A self-destructive nanosweeper that captures and clears amyloid β-peptides 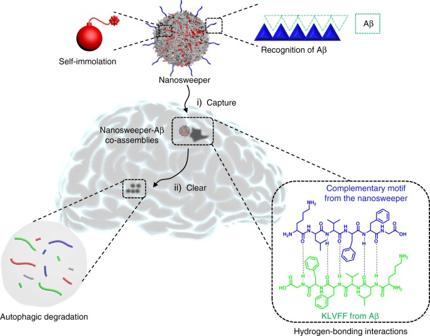Fig. 1 The schematic illustration of the nanosweeper mechanism of action. The nanosweeper captures Aβ by hydrogen-bonded co-assembly and internalizes a substantial amount into cells carrying Aβ. Then, the nanosweeper activates the cell’s autophagic response, resulting in the degradation of Aβ and the nanosweeper itself Cerebral amyloid β-peptide (Aβ) accumulation resulting from an imbalance between Aβ production and clearance is one of the most important causes in the formation of Alzheimer’s disease (AD). In order to preserve the maintenance of Aβ homeostasis and have a notable AD therapy, achieving a method to clear up Aβ plaques becomes an emerging task. Herein, we describe a self-destructive nanosweeper based on multifunctional peptide-polymers that is capable of capturing and clearing Aβ for the effective treatment of AD. The nanosweeper recognize and bind Aβ via co-assembly through hydrogen bonding interactions. The Aβ-loaded nanosweeper enters cells and upregulates autophagy thus promoting the degradation of Aβ. As a result, the nanosweeper decreases the cytotoxicity of Aβ and rescues memory deficits of AD transgenic mice. We believe that this resourceful and synergistic approach has valuable potential as an AD treatment strategy. Alzheimer’s disease (AD) has been considered the most pervasive neurodegenerative disorder, affecting a great number of humans worldwide [1] , [2] , [3] . The emphatic pathological hallmarks of AD are extracellular deposits of self-assembled fibrils based on the amyloid β-peptide (Aβ) and intracellular neurofibrillary tangles containing hyper-phosphorylated tau [4] , [5] , [6] , [7] , [8] . Over the past few decades, the trend in therapeutic methods for AD involved inhibiting the self-assembly of Aβ into fibrils and thus the resultant deposition of Aβ. Intense research indicates that inhibitors, such as antibodies [9] , peptide-based nanomaterials [10] , [11] , [12] , small molecules [13] , [14] , and various nanoparticles [15] , [16] , [17] , can decelerate the aggregation of Aβ. However, the recent failure of clinical trials based on bapineuzumab [18] and solanezumab [19] suggests that there is still a long way to go in treatment of AD against Aβ [20] , [21] . It has been accepted, when considering AD therapeutics, that the clearance of Aβ is the essential component in the maintenance of Aβ homeostasis. Autophagy, the way by which cells degrade their own metabolites, may be applied for Aβ clearance. Indeed, the dysfunction of the autophagy-lysosome system leads to the accumulation of Aβ [22] , [23] . It is beneficial for the enhancement of Aβ clearance that the induction of autophagy is appropriately elevated, giving rise to the distinct implication of autophagy as a therapeutic strategy [23] , [24] , [25] . However, because Aβ generated from amyloid precursor protein (APP) in endosomes is recycled to the cell surfaces and usually aggregates and deposits outside the cell while autophagic degradation occurs intracellularly, the concept of Aβ clearing by autophagy is contradictory. Herein, we design a nanosweeper with the goal of effectively degrading extracellular Aβ, and find that it not only captures extracellular Aβ and carries Aβ into cells, but it also up-regulates cellular autophagy and digestes Aβ. The nanosweeper is composed of a cationic chitosan (CS) core decorated with PEGylated-GKLVFF (designated as K) and Beclin-1 (TGFQGSHWIHFTANFVNT, designated as B). KLVFF can recognize and co-assemble with Aβ through hydrogen-bonding interactions. Beclin-1 can induce autophagy to degrade Aβ. The polyethylene glycol (PEG) increases the dispersity of the nanosweeper in water, providing the appropriate biocompatibility and stability. First, the nanosweeper captures and co-assembles with extracellular Aβ specifically, inhibiting the formation of toxic Aβ aggregates remarkably. Next, the nanosweeper preferentially delivers Aβ into cells and activates autophagy within them to degrade Aβ, ultimately resulting in Aβ clearance (Fig. 1 ). Results from in vitro and in vivo experiments confirms the nanosweeper’s high-efficiency for Aβ clearance. Among the Aβ-treated cells, the nanosweeper increases the cell viability from approximately 60 to 93%. Furthermore, the insoluble Aβ is decreased from 1539 to 914 ng/mg, and soluble Aβ is decreased from 585 to 190 ng/mg in the brain of AD transgenic mice treated with the nanosweeper, leading to rescued memory deficits. This delicate nano-strategy can be a potential therapeutic approach in the treatment of AD. Fig. 1 The schematic illustration of the nanosweeper mechanism of action. The nanosweeper captures Aβ by hydrogen-bonded co-assembly and internalizes a substantial amount into cells carrying Aβ. Then, the nanosweeper activates the cell’s autophagic response, resulting in the degradation of Aβ and the nanosweeper itself Full size image Preparation of the nanosweeper A series of nanosweepers with various chemical compositions were established by changing the peptide ratios [26] . There were two functional peptide analogs, a KLVFF peptide that could recognize and bind with Aβ 42 [27] , [28] , and a Beclin1 peptide that could significantly induce autophagy [29] , [30] . Both functional peptides were applied for linking with chitosan (CS) that was first modified by acrylate (acryl-CS). To control the hydrophobic/hydrophilic balance of the nanosweeper, PEG 368 was used to modify the G residue of the GKLVFF peptide. As shown in Fig. 2a , the feed molar ratios of KLVFF (Supplementary Fig. 1 ) and Beclin-1 were adjusted to obtain polymers with various peptide ratios. The final products were designated as M 1 , M 2 , M 3 , M 4 , and M 5 . The structures of acryl-CS and M 1–5 were confirmed by 1 H NMR. As shown in Fig. 2b , the 1 H NMR spectrum of acryl-CS revealed acrylate double bonds at 5.8–6.3 ppm. However, the acrylate double bonds in the 1 H NMR of M 1–5 disappeared entirely, indicating that the acrylate groups in acryl-CS reacted completely with sulfhydrylated KLVFF and Beclin-1 peptide. The peaks at 6.7–8.5 in the spectra of M 2 , M 3 , M 4 and M 5 were typical Beclin-1 peaks [30] . 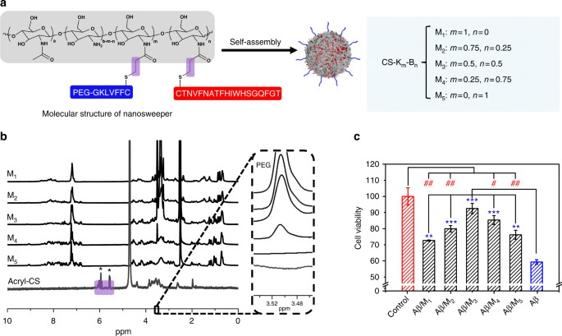Fig. 2 The molecular structure and biological effect of M3in vitro.aMolecular structures of the multifunctional peptide-polymer M1–5, K and B were the abbreviation of HS-CFFVLKG-PEG (capture unit) and HS-CTNVFNATFHIWHSGQFGT (clearance unit), respectively.bThe1H NMR of M1–5in6D-DMSO and acryl-CS in6D-H2O.cAβ cytotoxicity (20 μM) to N2a cells was reduced in the presence of 20 μg·mL−1M1–5. Data are presented as mean ± standard deviation (s.d.) (n= 3), analyzed by a Student’st-test. Statistical significance is indicated as *p< 0.05, **p< 0.01, and ***p< 0.001, for comparison with Aβ group,#p< 0.05,##p< 0.01, and###p< 0.001 for comparison with control group Meanwhile, a characteristic PEG peak appeared at 3.4–3.6 in the 1 H NMR spectra of M 1 , M 2 , M 3 and M 4 , but not in that of M 5 . Fig. 2 The molecular structure and biological effect of M 3 in vitro. a Molecular structures of the multifunctional peptide-polymer M 1–5 , K and B were the abbreviation of HS-CFFVLKG-PEG (capture unit) and HS-CTNVFNATFHIWHSGQFGT (clearance unit), respectively. b The 1 H NMR of M 1–5 in 6 D-DMSO and acryl-CS in 6 D-H 2 O. c Aβ cytotoxicity (20 μM) to N2a cells was reduced in the presence of 20 μg·mL −1 M 1–5 . Data are presented as mean ± standard deviation (s.d.) ( n = 3), analyzed by a Student’s t -test. Statistical significance is indicated as * p < 0.05, ** p < 0.01, and *** p < 0.001, for comparison with Aβ group, # p < 0.05, ## p < 0.01, and ### p < 0.001 for comparison with control group Full size image Biocompatibility and anti-Aβ toxicity of the nanosweeper In order to investigate the biological effects of the nanosweeper, we first explored its biocompatibility by measuring cytotoxicity in the mouse neuroblastoma cell line N2a. Cells were cultured with M 1–5 for 24 h, and then assessed by CCK-8 assay. As shown in Supplementary Fig. 2 , M 1–5 at a concentration of 20 μg·mL −1 showed good biocompatibility with approximate 100% viability, and so this concentration was utilized for further in vitro experiments. Next, to measure the anti-Aβ toxicity of M 1–5 , we detected the cell viability of N2a cells treated with Aβ 42 (20 μM) in the absence or presence of M 1–5 (20 μg·mL −1 ). As shown in Fig. 1c , Aβ 42 alone exhibited obvious toxicity (cell viability, 59.3%), which confimred the findings of previous reports [6] , [31] , [32] . However, adding nanosweepers reduced the toxicity of Aβ 42 . M 2–4 containing both K and B treated groups showed remarkably higher cell viabilities (* p < 0.05, ** p < 0.01, *** p < 0.001, Student’s t-test) than M 1 and M 5 treated groups, which only contains either K or B. This difference in cell viabilities indicated that the combination of both functional peptides resulted in a synergistic anti-Aβ - toxicity effect. M 3 showed the highest cell viability (92.5%), close to that of the control group (100%) and was screened as the potential lead nanosweeper for clearance of Aβ and AD treatment. To further verify the synergistic anti-Aβ toxicity effect of M 3 , two control peptide-polymers were prepared, M K , in which the Beclin-1 peptide was replaced by a control peptide without autophagy activation functionality, and M B , in which the KLVFF peptide was replaced by a KAAGG peptide without Aβ capture functionality (Supplementary Fig. 3 ). The chemical structures of both control peptide-polymers were also confirmed by 1 H NMR spectra (Supplementary Fig. 4 ). The cell viability results of M K (78.0%) and M B (80.9%) implied that they had lower anti-Aβ toxicity than M 3 (Supplementary Fig. 5 ), which indicated that the enhanced anti-Aβ-toxicity seen with M 3 originated from the synergistic effect of KLVFF and Beclin-1. Capture of Aβ 42 by the nanosweeper In order to study the ability of the nanosweeper to regognize and co-assemble with Aβ 42 , we first employed the Thioflavin T (ThT) fluorescence assay to detect Aβ fibril formation in the presence of M 3 . The ThT assay, an established method of dye binding, was applied to monitor Aβ 42 aggregation because its fluorescent spectrum can be altered with the growth of fibrils [6] . 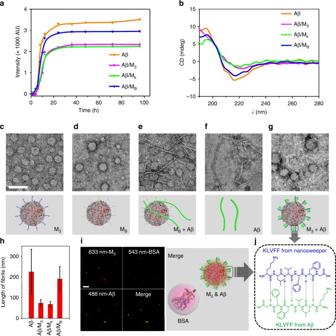Fig. 3 The capture of Aβ by M3through co-assembly.aThT fluorescence assay of Aβ and Aβ/M3in 96 h, with Aβ/MKand Aβ/MBas controls. Data are presented as mean ± s.d. (n= 3).bThe CD spectra of Aβ and Aβ/M3at 24 h, with Aβ/MKand Aβ/MBas controls.c–gTEM images of M3, MB, Aβ/MB, Aβ and Aβ/M3at 24 h.hThe statistical length of Aβ fibers was averaged from 5 individual fibers per group. Data are presented as mean ± s.d. (n= 5).iCLSM images and schematic illustration of the mixture of Cy5-labeled M3, FITC-labeled Aβ and Cy3.5-labeled BSA.jThe schematic illustration of the driving force for the capture of Aβ by hydrogen bonds. Scale bar: white bar in (c) is 100 nm, and (i) is 20 µm Figure 3a displays a series of sigmoidal curves which are typical of Aβ 42 fibrillation. The fluorescence intensity of neat Aβ 42 was higher due to the larger amount of Aβ 42 fibrillation formation than that of Aβ 42 in the presence of M 3 , which was similar to the result observed with M K , and much lower than that observed with M B. The decreasing ThT fluorescence seen from M 5 to M 1, together with the increasing KLVFF content (Supplementary Fig. 6 ), validated the recognition and co-assembly functionality of KLVFF, resulting in the inhibition of Aβ 42 aggregation. Furthermore, the results of circular dichromism (CD) spectra confirmed that M 3 inhibited the formation of β-sheet structrured Aβ 42 fibrils (Fig. 3b ). The Aβ 42 showed random structures at 0 h (Supplementary Fig. 7 ) and typical β-sheet structure at 24 h, with positive and negative signals at 195 and 216 nm, respectively. The M 3 or M K treated Aβ did not show typical β-sheet structures at 24 h, however, the M B treated Aβ 42 did show typical β-sheet structures at 24 h. The CD measurements also revealed the inhibitory effect of Aβ 42 fibrillation due to KLVFF recognition and co-assembly. Fig. 3 The capture of Aβ by M 3 through co-assembly. a ThT fluorescence assay of Aβ and Aβ/M 3 in 96 h, with Aβ/M K and Aβ/M B as controls. Data are presented as mean ± s.d. ( n = 3). b The CD spectra of Aβ and Aβ/M 3 at 24 h, with Aβ/M K and Aβ/M B as controls. c – g TEM images of M 3 , M B , Aβ/M B , Aβ and Aβ/M 3 at 24 h. h The statistical length of Aβ fibers was averaged from 5 individual fibers per group. Data are presented as mean ± s.d. ( n = 5). i CLSM images and schematic illustration of the mixture of Cy5-labeled M 3 , FITC-labeled Aβ and Cy3.5-labeled BSA. j The schematic illustration of the driving force for the capture of Aβ by hydrogen bonds. Scale bar: white bar in ( c ) is 100 nm, and ( i ) is 20 µm Full size image To provide evidence for supporting the binding effect of M 3 to Aβ 42 , transmission electron microscopy (TEM) and dynamic light scattering (DLS) were exploited to detect the evolution of morphology and size distribution in an Aβ 42 solution in the presence of M 3 , with M B and M K acting as control groups. The M 3 , M B, and M K in solution (H 2 O:DMSO = 98:2, 20 μg·mL −1 ) showed similar particulate structures with 43.8 ± 11.1 nm diameter at 24 h (Fig. 3c, d and Supplementary Fig. 8a ), and their surfaces could be composed by relative hydrophilic PEG 368 -GKLVFF (or PEG 368 -GKAAGG). Following a 24 h incubation with Aβ 42 at 37 °C, TEM images showed that Aβ 42 incubated with M B clearly contained separate morphologies of nanoparticles and nanofibers (Fig. 3e ) at 24 h, which were potentially originated from M B and Aβ 42 (Fig. 3f ), respectively. However, the Aβ 42 incubated with M 3 and M K contained main species of particulate structures entangled with some fibers (Fig. 3g and Supplementary Fig. 8b ), the morphology of which was totally different from free mature Aβ 42 fibrils. Interestingly, the statistics obtained from the fiber length taken from the TEM images of Aβ 42 , and Aβ 42 /M B showed similar lengths, 225 ± 109 and 191 ± 60 nm (Fig. 3h ), respectively. The statistical length of Aβ 42 /M 3 and Aβ 42 /M K was decreased to 74 ± 17 and 68 ± 13 nm, respectively, suggesting that M 3 and M K could co-assemble with Aβ 42 and inhibit the formation of free mature Aβ 42 fibrils, probably through KLVFF recognition and binding unit. These TEM results were in accordance with the DLS measurement (Supplementary Fig. 9 ). Confocal laser scanning microscopy (CLSM) was further employed to validate the specific co-assembly of Aβ 42 and M 3 . We first labeled M 3 nanosweeper and Aβ 42 with Cy5 (M 3 -Cy5) (Supplementary Fig. 10 ) and FITC (Aβ 42 -FITC), respectively. The M 3 -Cy5 and Aβ 42 -FITC were mixed in water and co-localized well by CLSM measurement, so was M K -Cy5 with Aβ 42 -FITC (Supplementary Fig. 11 ). However, there were no obvious co-localization observed between M B -Cy5 and Aβ 42 -FITC, indicating that the KLVFF induced the co-assembly of M 3 /M K and Aβ 42 . In order to confirm the specificity, Cy3.5-labeled bovine serum albumin (BSA), a kind of serum albumin, accoutning for 55% of blood proteins, was utilized as a competing regent. The M 3 -Cy5, Aβ 42 -FITC, and BSA-Cy3.5 were mixed together, and observed by CLSM. The results clearly displayed that the M 3 -Cy5 co-localized with Aβ 42 -FITC, but not BSA-Cy3.5, providing strong evidence for the specific co-assembly between M 3 -Cy5 and Aβ 42 -FITC (Fig. 3i,j ). Delivery of Aβ 42 into cells by the nanosweeper To confirm that the Aβ 42 was substantially internalized into neutron cells by M 3 , N2a cells in a confocal petri dish (20 mm) were treated with Aβ 42 -FITC (20 μM), M 3 -Cy5, M K -Cy5, M B -Cy5 (20 μg·mL −1 ) and a mixture of Aβ 42 -FITC/M 3 -Cy5, Aβ 42 -FITC/M K -Cy5, Aβ 42 -FITC/M B -Cy5 and observed by CLSM (Fig. 4 ). As can be seen in Fig. 4 , the Aβ 42 -FITC treated N2a cells exhibited green signal on cell surfaces, but not in the cytoplasmic matrix. This finding indicated that Aβ 42 might get stuck in the membrane during internalization into cells, due to its hydrophobicity, which most likely led to neurotoxicity in the N2a cells. Nanosweepers, such as M 3 -Cy5, M K -Cy5, and M B -Cy5 were internalized into cells with red fluorescence in cytoplasm (Supplementary Fig. 12 ). As expected, N2a cells treated with Aβ 42 -FITC/M 3 -Cy5 showed green Aβ 42 -FITC fluorescence co-localized with M 3 -Cy5 (Pearson’s correlation coefficient (PCC) = 0.72) inside cells, due to the capture of Aβ 42 by the M 3 nanosweeper and the subsequent high-efficiency internalization into cells (Fig. 4 ). M 3 increased the internalization of Aβ 42 through co-assembly, not attaching on cell surfaces. The positive control group cells that were treated with Aβ-FITC/M K -Cy5 displayed the colocalized fluorescence of Aβ 42 -FITC and M K -Cy5 inside cells with PCC of 0.67, similar to the Aβ 42 -FITC/M 3 -Cy5 group. However, the group treated with Aβ 42 -FITC/M B -Cy5 (PCC = 0.44) showed red fluorescence (M B -Cy5) inside cells and merged Aβ 42 -FITC and M B -Cy5 on cell surfaces (Supplementary Fig. 13 ). These results suggested that M B entered the cells alone, and that the Aβ 42 -FITC stuck on cell surfaces as usual. When cell surfaces were covered with Aβ 42 -FITC, the M B -Cy5 may no longer be able to enter cells, but stayed on cell surfaces, showing the merged fluorescence signals on cell surfaces. Therefore, the co-assembly of M 3 and Aβ 42 not only inhibited the Aβ 42 fibril formation, but also increased the internalization of Aβ 42 . Fig. 4 Aβ was internalized into cells with M 3 nanosweeper. Schematic (row 1) and CLSM measurements of N2a cells treated with Aβ, a mixture of Aβ/M 3 , Aβ/M K and Aβ/M B (row 2, 633 nm; row 3, 488 nm; row 4, Merge). Scale bar: 20 µm Full size image Inducement of autophagy by the nanosweeper in vitro In order to validate the autophagy effect of M 3 on N2a cells, autophagic structures and the marker protein LC3-II were measured using Acridine Orange staining, Bio-TEM, and western blot methods. Acridine Orange (AO) is a pH-sensitive dye and typically used as non-specific chemical agent for autophagy detection. It can mark acidic vesicular organelles with red and cytoplasm and DNA with green [30] . The ratio of red/green has been used widely to evaluate levels of autophagy [33] , [34] . The N2a cells were incubated with M 3 , and M B and M K as controls for 4 h, then stained with AO dyes for 10 min, followed by observation by CLSM. As shown in Supplementary Fig. 14a , there were many red spots in the M 3 -treated and M B -treated cells. In contrast, PBS and M K treated cells showed few red spots. The quantification of fluorescence revealed that the red/green signal ratios of the M 3 -treated and M B -treated groups were remarkably higher than those of the PBS-treated and M K -treated cells (Supplementary Fig. 14b , *** p < 0.001). In addition, bio-TEM, a standard method for autophagy detection, was applied to examine the autophagic structures (autophagosome and autolysosome) of N2a cells. The N2a cells were first treated with M 3 , M K and M B for 4 h, after which the cells were harvested and prepared for bio-TEM imaging using our previous method [35] . Finally, a JEOL JEM-1400 electron microscope was used to observe cells. As shown in Fig. 5a , an increase in the amount of small double/multi-membrane vesicles (autophagosome, black arrow) and huge vacuoles (autolysosome, white arrow) were observed in the M 3 -treated and M B -treated cells, compared with the PBS group. However, there were minimal autophagic structures in the M K -treated cells. The statistic results showed dramatic differences between M K and M 3 treated groups (Fig. 5b , * p < 0.05 Student’s t -test). In addition, the results of western blotting for LC3-II, an autophagy marker protein, confirmed that M 3 increased the expression of LC3-II significantly (Fig. 5c, d ). The above results lent strong support to the hypothesis that Beclin-1 residues in M 3 could effectively induce autophagy in vitro. Fig. 5 M 3 activated autophagy significantly in vitro. a TEM images of N2a cells. The N2a cells were treated with PBS (control), M K (200 μg/mL) and M 3 (200 μg/mL), and M B (200 μg/mL). The autophagic structures are indicated by black arrows (autophagosome), and white arrows (autophagic vacuoles). b The static results of autophagic structures were obtained from three random TEM images. Data are presented as mean ± s.d. ( n = 3). c Western blot of LC3-II and ( d ) the corresponding quantified results. N2a cells were treated for 24 h with PBS (control), M K (200 μg/mL), M 3 (200 μg/mL), and Rapa (1 μM). Data are presented as mean ± s.d. ( n = 3). Statistical significance is indicated as * p < 0.05, ** p < 0.01, and *** p < 0.001, for comparison with control group (Student’s t -test) Full size image Autophagic degradation induced by the nanosweeper in vitro We studied the autophagic flux of N2a cells in order to explore whether or not intracellular M 3 &Aβ 42 adduct could be degraded by the autophagic process. M 3 was first labeled with Cy5 (red signal). Next, the GFP-LC3 transfected N2a cells were incubated with M 3 -Cy5&Aβ 42 (20 μg·mL −1 /20 μM) for 4 h, followed by CLSM observation. Generally, LC3-II was recruited to the autophagosome membrane and thereby formed a green dot of GFP-LC3 when autophagy was activated [36] , [37] . As expected, the CLSM images revealed that most of the M 3 -Cy5 (red signal) colocalized with autophagosomes (GFP-LC3, green signal) (Fig. 6a ), indicating that M 3 &Aβ 42 was delivered to autophagosomes. Generally, the autophagosome would be fused with the lysosome, forming an autolysosome for degredation of cargo [38] . 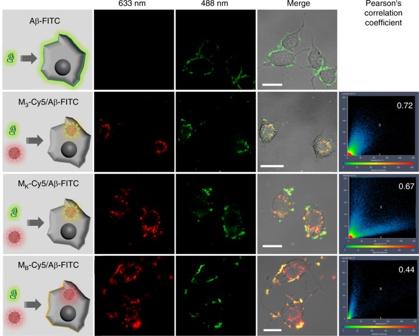Fig. 4 Aβ was internalized into cells with M3nanosweeper. Schematic (row 1) and CLSM measurements of N2a cells treated with Aβ, a mixture of Aβ/M3, Aβ/MKand Aβ/MB(row 2, 633 nm; row 3, 488 nm; row 4, Merge). Scale bar: 20 µm So, we therefore measured the colocalization of M 3 -Cy5&Aβ 42 with autolysosomes. p62, An autolysosome marker protein that is preferentially degraded by autophagic process, was marked with green fluorescence through an immunofluorescence technique. The results displayed that the green immunofluorescence signals from p62 and red fluorescence signals from M 3 -Cy5 were highly merged (Fig. 6b ), indicating that M 3 &Aβ 42 was transferred into the autolysosome for degradation (Fig. 6c ). To further confirm autophagic degradation, we used western blotting to detect the autophagic flux based on expression of p62. As shown in Fig. 6d , M 3 upregulated the expression of p62, similarly to HCQ and Rapa. However, M 3 did not induce obvious p62 upregulation of the Rapa-treated group, but increased accumulation of p62 in the HCQ-treated group, with a p62/β-actin ratio from 2.58 to 3.10 (Fig. 6e ). These findings validated that M 3 activated autophagy without blockade of the autophagic flux, indicating the possibility of autophagic degradation of Aβ 42 . Fig. 6 M 3 induced autophagic degradation in vitro. a CLSM images showed the co-localization of the autophagosome (GFP-LC3-positive puncta, green signals) and M 3 -Cy5 (red signals). N2a/GFP-LC3 cells were treated with M 3 -Cy5 (200 μg/mL) and M K -Cy5 as a control for 24 h. b CLSM images showed the co-localization of M 3 -Cy5 (red signals) and p62 (green signals from anti-p62-labeled secondary antibody). c The schematic illustration of M 3 degradation by autophagy. d Western blot of p62 and ( e ) the corresponding quantified results. N2a cells were cultured as follows: in regular culture medium for 24 h (lane 1); M 3 (200 μg/mL) for 24 h (lane 2); 5 μM HCQ for 1 h (lane 3); 1 μM Rapa for 1 h (lane 4); with M 3 (200 μg/mL) and HCQ (lane 5); with M 3 (200 μg/mL) and Rapa (lane 6); with Rapa and HCQ (lane 7). Data are presented as mean ± s.d. ( n = 3). Scale bar in ( a , b ) is 10 µm Full size image Crossing BBB and activating autophagy in vivo For the in vivo experiment, the nanosweeper should be effectively delivered into brain. Cyclosporine was verified to effectively increase the permeability of blood-brain barrier (BBB) through influencing P-gp function in the BBB [39] , [40] . In order to evaluate how M 3 nanosweeper crossed the BBB, we intravenously injected cyclosporine (10 μM) into mice, followed by i.v. administration of a dose of 200 μg·mL −1 M 3 nanosweeper, which was labeled by Cy5. The mice were sacrificed and the brains were harvested for ex vivo imaging. As shown in Supplementary Fig. 15 , the higher fluorenscence signal in cyclosporine and M 3 -Cy5 nanosweepers indicated that cyclosporine made more M 3 nanosweepers reaching to the brain, compared with PBS or M 3 -Cy5 nanosweeper treated group. Furthermore, for quantifying the efficiency of M 3 nanosweepers crossing BBB, we loaded the very small gold NPs into M 3 nanosweepers, and i.v. injected into the mice 30 min after cyclosporine i.v. administration. The M 3 nanosweepers distribution in the brain was characterized by gold amount, which was measured by inductively coupled plasma mass spectrometry. M 3 nanosweepers reaching the brain could be calculated as 1.94% of total injection (Fig. 7a ). Fig. 7 In vivo evaluation of M 3 crossing BBB and activating autophagy. a The concentration of Au in the brain and in the total injection solution, respectively. The amount of M 3 actually reached to the brain was evaluated by Au amount: M 3 % = 0.03/1.55 × 100% = 1.94%. ( n = 4). b CLSM images and c bio-TEM images of brain tissue slices of AD mice treated by PBS or M 3 , and WT mice treated with PBS as a control. The dots of GFP-LC3 (white arrow in b ) and the strucuture of autophagsome (black arrow in c ) were pointed out in M 3 treated AD mice, respectively. Scale bar in ( b ) is 20 µm. Scale bar in ( c ) is 1 µm Full size image The activation of autophay in the brain determined the therapeutic effect, the immunohistochemical method was utilized for confirming the autophagic process of hippocampal neuron activated by M 3 nanosweepers. Sections of the hippocampi from mice were stained with LC3 antibody marked with FITC. The CLSM images displayed an increased dots of green signals (autophagic structures) in the M 3 -treated mice than that of the wild type (WT) and AD groups (Fig. 7b ), indicating the more LC3, the biomarker of autophagy in M 3 treated mice brain. In addition, brain slices of AD mice treated with M 3 were observed by bio-TEM, and the results were shown in Fig. 7c . There were a lot of autophagic structures in M 3 treated group, but not observed in WT and AD groups without treatment. These results suggested that M 3 could effectively induce the autophagic process in vivo. Clearance of Aβ and rescue of memory deficits In order to further study whether or not the M 3 nanosweeper could reduce amyloid plaques in the brains of AD mice, M 3 nanosweeper was utilized to treat APPswe/PS1dE9 transgenic mice every other day for one month [15] , [16] , [41] . Following the treatment period, the amount of soluble Aβ 42 and insoluble Aβ 42 in the brain tissue was measured by enzyme-linked immune sorbent assay (ELISA) (Fig. 8a,b ), and confirmed that soluble Aβ 42 and insoluble Aβ 42 were decreased by M 3 treatment, which was obvious lower than those of AD mice without treatment. As expected, M 3 nanosweeper may capture Aβ 42 to form M 3 and Aβ 42 and enter into cells, followed by activation of autophagy and degradation of Aβ 42 intracellluarly, leading to the decrease of soluble Aβ 42 . The decrease of soluble Aβ 42 further resulted in the decrease of Aβ 42 aggregation, i.e., insoluble Aβ 42. Furthermore, immunohistochemistry analysis was carried out to label Aβ deposition in the brains. As shown in Fig. 8c , a large amount of Aβ deposition (circled with red dotted line) was observed in the AD control mice, and the difference was obvious between those and the WT control mice. Importantly, in the brains of AD mice treated with M 3 nanosweeper, there was a significant decrease in the Aβ plaque load, indicating that M 3 nanosweeper had the ability to reduce Aβ deposition, which was in agreement with the measurments of Aβ in the brain. The soluble and insoluble Aβ in the brain of AD mice treated with M 3 was also decreased (Supplementary Fig. 16 ), but not as much as the extend of decrease in Aβ 42 , probably indicating the specificity of M 3 for capture of Aβ 42 by KLVFF. The results of Nissl staining of nerve cells revealed an obvious neuronal hypocellularity in the brain of AD control mice, which had small amounts of Nissl bodies (blue) (Fig. 8d ). Contrastingly, M 3 nanosweeper treatment significantly attenuated neuron loss in AD mice. Together, these results indicated that M 3 nanosweeper could effectively decrease soluble Aβ 42 and insoluble Aβ 42 , as well as the the deposition of Aβ and toxicity in nerve cells. Fig. 8 In vivo evaluation of M 3 for the clearance of Aβ and decreasing cytotoxicity. a Soluble Aβ 42 and ( b ) insoluble Aβ 42 in the brain measured by ELISA. ( n = 4). c The immunohistochemical analysis of Aβ 42 deposition in the brains of WT control mice, AD control mice, AD mice treated with M 3 . The Aβ 42 deposits appeared as brown signals as indicated by red dotted circle. Scale bar is 50 µm. d The Nissl staining of nerve cells in the brains of WT control mice, AD control mice, AD mice treated with M 3 . The Nissl bodies were stained blue. Scale bar is 50 µm. e The latencies of WT control mice, AD control mice, and AD mice treated with M 3 (three mice per group). f The latency during the memory test in the MWM probe trial without a platform. g The percent (%) of time in the targeted quadrant where the platform had been located during the memory test in the MWM probe trial. h , i were the quantified results of ( c , d ), respectively. Data are presented as mean ± s.d. ( n = 6). The data between AD group and M 3 group are analyzed by a Student’s t -test. Statistical significance is indicated as * p < 0.05, ** p < 0.01, and *** p < 0.001 Full size image The Morris water maze (MWM) test was utilized to investigate the effect of M 3 nanosweeper on the spatial cognitive performance of APPswe/PS1dE9 transgenic mice. The escape latencies of M 3 -treated mice for searching for the hidden platform were measured daily for 4 days. As shown in Fig. 8e , both WT mice and M 3 nanosweeper-treated AD mice exhibited significantly shorter latency than the AD control group on days 2, 3, and 4, indicating that M 3 nanosweeper could markedly improve the spatial memory of AD mice. When the training was completed, the place of the platform was removed and the mice were given 60 s to find the missing platform for the probe trial. As shown in Fig. 8f , the M 3 nanosweeper-treated AD mice exhibited spatially oriented swimming behavior and shorter latencies than AD control mice. These outcomes were further confirmed by the percentage of time spent in the target quadrant (Fig. 8g ). The number of times M 3 nanosweeper-treated mice entered the small target zone was 2.4, which was greater than that of the AD mice (1.6 times). In order to evaluate long-term therapetuic effect, M 3 nanosweeper was utilized to treat APPswe/PS1dE9 transgenic mice every other day for one month, and the MWM was tested two month post-treatment. The searching ability for the hidden platform of AD mice treated with M 3 nanosweeper was obviously enhanced (Supplementary Fig. 17 ), similar as the above results, revealing that the excellent long-term therpeutic effects of M 3 nanosweeper. The systemic toxicity of M 3 was further investigated by hematology and histopathology assays (Supplementary Figs. 18 and 19 ). No significant differences were detected in pathological signs (heart, liver, spleen, lung, and kidney) between the M 3 -treated group and the control groups (WT and AD). All of above results suggested that M 3 did not cause any obvious side effects and could be used safely as a biomaterial with excellent rescue of memory deficits in AD transgenic mice. In summary, we successfully developed a multifunctional peptide-polymer based nanosweeper (M 3 ), which could specifically capture Aβ via recognition and co-assembly with Aβ, followed by delivery of Aβ into cells. The nanosweeper promoted degradation of Aβ through the upregulation of autophagy. Both in vitro and in vivo experiments were performed to validate this hypothesis and the remarkable resulting anti-AD therapeutic effect. M 3 increased the cell viability of N2a cells, which was induced by Aβ. Moreover, M 3 decreased Aβ deposition in the brains of APPswe/PS1dE9 transgenic mice and rescued their memory deficits. The nanosweeper could have clinical practicality and provide an efficient therapeutic system for clearance of Aβ. Collectively, our findings support the potential for this new multifunctional peptide-polymer, the nanosweeper, as an promising therapeutic agent for the treatment of AD, opening up a new avenue for therapeutic applications. Materials Chitosan (CS, average Mw 5000), acryloyl chloride (TCI, Shanghai, China), Methoxy poly(ethylene glycol) (CH 3 O-PEG n -CH 2 CH 2 COOH) (M n = 368) was purchased from Jiaxing Biomatrix and Biotechnology Inc. Thioflavine-T, Cy3.5 and Cy5 were obtained from Sigma-Aldrich. 1,1,1,3,3,3-Hexafluoro-2-propanol (HFIP) and dimethyl sulfoxide (DMSO) were purchased from Aldrich Chemical Co. and used without further purification. Aβ, FITC-Aβ, Beclin-1 (B) (>95%) and scrambled Beclin-1 peptide (B’) (>95%) were customized from GL Biochem Ltd. (Shanghai, China). Aβ 42 was pre-treated with HFIP, followed by evaporation with N 2 and stored at −20 °C. Cell counting kit-8 assay (CCK-8) (Beyotime Institute of Biotechnology, China) were used without further purification. Other solvents and reagents were used as received. Preparation of peptides Firstly, acryl-CS was obtained as our previous reports. Peptide CFFVLKG-PEG (abbreviate to K) and CGGAAKG-PEG (abbreviate to K’) were prepared by standard solid phase peptide synthesis techniques using F moc -coupling chemistry. Acryl-CS (0.021 g, 0.1 mM for acrylamide bonds) was dissolved in PBS solution (2.1 mL, pH 8.0), 0.12 mM peptides in total with different ratio of m/n (1:0, 0.75:0.25, 0.5:0.5, 0.25:0.75, 0:1) were dissolved in 2.1 mL DMSO, followed by dropwise addition into acryl-CS solution under magnetic stirring. Then, the mixtures were bubbled with N 2 for 30 min under stirring and reacted at 37 °C for 48 h in the dark. After the reaction, the resultant solution was dialyzed against deionized water (MWCO: 3500 Da) for 24 h and lyophilized to obtain a pale yellow solid. M K (CS-K 0.5 -B’ 0.5 ) and M B (CS-K’ 0.5 -B 0.5 ) were obtained by the same method. Characterization of peptides The CFFVLKG-PEG and CGGAAG-PEG were confirmed by matrix-assisted laser desorption ionization time-of-flight mass spectrometry (MALDI-TOF-MS, Bruker Daltonics). The chemical structures of M 1–5 , M K , and M B were proven by NMR measurements. 1 H NMR spectra (400 MHz) of the M 1–5 , M K , and M B in d 6 -H 2 O and Acryl-CS in d 6 -DMSO were recorded on a Bruker ARX 400 MHz spectrometer. ThT fluorescence assay The ThT fluorescence assay was recorded at 485 nm through microplate absorbance reader (Tecan infinite M200, Switzerland) with excitation wavelength of 450 nm. For each measurement, the pre-treated Aβ solutions with and without M 1–5 , M K , and M B were co-incubated with ThT solutions in phosphate buffer to the final concentration of Aβ peptide at 20 μM, M 1–5 , M K , and M B at 20 μg·mL −1 , ThT at 20 μM. Circular dichroism (CD) spectra The CD spectra of Aβ (0.09 mg·mL −1 , 20 μM) with or without M 3 , M K , and M B (20 μg·mL −1 ) were monitored using a CD spectrometer (JASCO-1500, Tokyo, Japan) with a cell path length of 1 mm at room temperature. The measurements were implemented between 190 nm to 280 nm with a resolution of 1.0 nm and a scanning speed of 300 nm·minute −1 . For each measurement, 3 spectra were collected and averaged. Transmission electron microscopy (TEM) The morphologies of M 3 , M K , and M B nanoparticles, Aβ fibril and their mixture were observed by TEM (Tecnai G2 20 S-TWIN) with an acceleration voltage of 200 kV. The M 3 , M K , and M B nanoparticle solutions were prepared by dispersing 5 mg·mL −1 DMSO into PBS with a final concentration of 20 μg·mL −1 . The Aβ nanofibril (20 μM) and the co-assembly solutions were obtained after incubating 24 h at 37 °C. 10 μL of the solutions were dropped onto a copper mesh for 5 min, subsequently removed most of the liquid through a filter paper. 10 μL of uranyl acetate solution was employed to stain the samples for 5 min, followed by drying the spare liquid with the filter. Finally, the copper mesh was washed with 10 μL of deionized water, which was blotted after staining and dried at room temperature. Cytotoxicity assay for mouse neuroblastoma N2a cells Mouse neuroblastoma N2a cell line was purchased from cell culture center of Institute of Basic Medical Sciences, Chinese Academy of Medical Sciences (Beijing, China), and was utilized to evaluate the cytotoxicity of M 1–5 , M K , and M B nanoparticles by the CCK-8 assay. A density of 5 × 10 3 N2a cells per well were seeded in the 96-well plates in DMEM supplemented with 10% fetal bovine serum (FBS) and 1% penicillin-streptomycin in a humidified atmosphere with 5% CO 2 and then cultured at 37 °C for a night. 10 μL of M 1–5 , M K , and M B were dispersed in DMEM medium with a series of different concentrations, 10, 20, 50, 100, 200 μg·mL −1 to obtain an optimal M 1–5 , M K and M B concentration. Aβ at the concentration of 20 μM with and without M 1–5 , M K and M B sample solutions were co-incubated with cells for additional 24 h. Subsequently, 10 μL of CCK-8 solutions was added to each well and cultured for 4 h. The UV-vis absorptions of sample wells (A sample ), A blank and control wells (A control ) were performed by a Microplate reader at a test wavelength of 450 nm and a reference wavelength of 690 nm, respectively. Cell viability (%) was equal to (A sample − A blank )/(A control − A blank ) × 100%. All the experiments were performed in triplicate. The cell lines had been authenticated utilizing short tandem repeat DNA profiling. All cells were tested negative for cross-contamination of other human cells and mycoplasma contamination. Confocal laser scanning microscopy (CLSM) observation The N2a cells incubated with and without M 3 , M K , and M B were investigated on a Zeiss LSM710 confocal laser scanning microscope (Jena, Germany). N2a cells were seeded in complete DMEM media in a humidified atmosphere with 5% CO 2 and then cultured at 37 °C for a night. For co-localization analysis, the medium was replaced by 1 mL of serum free fresh medium containing 20 μg (M 3 , M K , and M B ) Cy5-labeled nanoparticles, 20 μM FITC-labeled Aβ. Then the cell were cultured with the serum free fresh medium for another 2 h and washed with PBS for 3 times. After replacement of the medium with PBS, cells were imaged using a Zeiss LSM710 confocal laser scanning microscope with a ×63 objective lens. Western blotting analysis N2a cells were treated with M 3 , M K and M B (20 μg·mL −1 ) for 12 h, and then re-suspended lysis buffer solution with 1% (v/v) Triton-X 100 in 150 mM NaCl and 50 mM Tris-HCl (pH = 8.0). The protein content was estimated by a BCA kit (Applygen). Each sample (60 μg of protein) was subjected to SDS-PAGE and then transferred to a nitrocellulose membrane. Blots were blocked in a blocking buffer containing 5% (wt/v) non-fat milk, 0.1% (v/v) Tween 20 in 0.01 M TBS, and incubated with primary antibodies overnight at 4 °C and then incubated with an appropriate secondary antibody (ZSGB-BIO) for another hour at room temperature, subsequently scanned on a Typhoon Trio Variable Mode Imager. Band density was calculated using ImageJ software. The following antibodies were used: LC3B (AL221, 1:1000 dilution, Beyotime Institute of Biotechnology, China), β-actin (30101ES, 1:1000 dilution, Yeasen Biology Ltd., China) and p62 (5114, 1:1000 dilution, CST). Uncropped blots were presented in Supplementary Fig. 20 . Bio-TEM for autophagy in vivo The part of brain from mice were first fixed overnight at 4 °C in PBS buffer with 2.5% glutaraldehyde. After washing with PBS buffer (0.1 M) for three times, the brain tissues were fixed at room temperature with 1% osmium-containing PBS buffer for 2 h. Subsequently, all the brain tissues were washed three times with PBS buffer and dehydrated with a graded series of acetone (50, 70, 80, 90, 95, 100%) for 15 min for each step. After infiltrated with a graded of series of mixtures (acetone/EPON 812 resin: 2/1, 1/1, 1/2) at room temperature for 1 h, pure resin was added and incubated overnight at 4 °C. Finally, the gelatin capsules were used to cover the tissues and incubated with pure EPON 812 resin at 37, 45, and 60 °C for 24 h, respectively. The tissues were cut into ultrathin sections by a diamond knife and picked up with Formvar-coated copper grids (300 mesh). All of the sections were performed counter-staining with osmic acid (1%) for 1 h and uranyl acetate (4%) for 20 min, respectively. JEOL JEM-1400 electron microscope (JEOL, Tokyo, Japan) was used to observe tissues. Measurement of soluble and insoluble Aβ 42 in the brain Brain tissue (one brain hemisphere, 4 mice per group) for ELISAs was mechanically homogenized in 10 volumes of ice-cold guanidine buffer pH 8.0) and were mixed for 3 to 4 h at room temperature (RT) as described [42] . Then diluted brain homogenates with 1:10 by ice-cold casein buffer (0.25% casein/0.05%sodium azidey/20 mg/mL aprotininy/5 mM EDTA, pH 8.0/10 μg/mL leupeptin in PBS) was centrifuged 30 min at 4 °C for 16,000× g . The supernatant included 0.5 M guanidine in the presence of 0.1% bovine serum albumin (BSA) was removed for ELISA measurement for soluble Aβ 42 and Aβ total or stored −80 °C. The homogenate pellet that remains after centrifugation were added 425 µL cold formic acid and kept tubes on ice. Each sample was sonicated on ice continuously until that the pellet dissolved. Then performed high-speed spin at 109,000× g for 1 h at 4 °C and took 105 µL sample and add 1.895 mL of formic-acid neutralization buffer (1 M Tris base/0.5 M Na 2 HPO 4 /0.05% NaN 3 ) on ice for ELISA measurement for insoluble Aβ 42 and Aβ total or stored −80 °C. Mouse Aβ 1–42 ELISA Kit (R141671) and Mouse Aβ ELISA Kit (R167250) from the Trust Specialty Zeal biological trade Co., Ltd., U.S.A. were used, respectively. Morris water maze (MWM) experiment Animal experiments were carried out complying with NIH guidelines for the Care and Use of Laboratory Animals, and the study the protocol was approved by the Institutional Animal Care and Use Committee of National Center for Nanoscience and Technology, China. All animals were obtained from Beijing HFK bioscience Co., Ltd. (Beijing, China). The non-Tg C57 mice were regarded as wild type mice (WT mice). The APPswe/PS1dE9 transgenic mice (AD mice) were divided into two group, AD group and M 3 group (3 mice per group). All mice were male, and 9 month old, which intravenously administered PBS and M 3 nanoparticles, respectively. All mice were trained and tested in a water maze with a diameter of 1.1 m. The maze was filled with water and drained daily. The temperature of the water was maintained at 22 ± 1 °C. The platform (0.1 m in diameter) was immobilized to 1 cm under the water surface during the training period, whereas the starting points were counter balanced. From the first day to the fourth day during training, the mice were measured four times from four diversed positions around the border of the maze in a semi-random order with 60 s latent period to reach the platform. If the animal find the hidden platform successfully within 60 s, it was allowed to stay on the platform for 15 s. If it failed to find the platform, the mice had to be placed on the platform for 15 s. The motional orbits of each mice was recorded and studied using a computerized video-tracking system. When the last learning trial was finished, the memory capacity of each mice were explored by a probe trial without the platform. Every trained animal was allowed to swim freely for 60 s, with two initial sites far away from the targeted platform. The time each mouse spent in searching for the platform in the quadrant where the platform used to be (target quadrant), and the number of times it crossed the target quadrant was recorded. Immunohistochemical analysis and nissl staining After the MWM test, the mice were euthanized. The tissue sections in the coronal plane at 40 µm on a freezing sliding microtome from the genu of the corpus callosum through the caudal extent of the hippocampus (3 µm-thick, 4 sections/mouse, 3 mice/group). For qualitative analysis of Aβ immunoreactivity, half sections were immunostained as described [43] with the following Aβ antibodies: Rabbit Anti-beta-Amyloid 1–42 (CT antibody) (bs-0076R, 1:200, Bioss, Beijing, China) and Anti-rabbit IgG (H + L) Aβ Hrp (074-1506, 1:200, KPL, Massachusetts, USA). The sections were observed under a microscope (XSP-C204, COIC, China). Pictures were acquired with a digital camera and analyzed with the ImageJ software. The area occupied by Aβ plaques was quantified as the percent surface area occupied in the delineated hippocampus. The plaques were quantified as the ratio of plaques vs corresponding hippocampal area and the detailed process was shown as follows: The ratio of plaques vs hippocampal area (R%) was calculated based on R% = S t /S × 100%. S t is the total area of plaques, and the S t = S 1 + S 2 + S 3 + …, where the S 1 , S 2 , S 3 … indicates the area of each plaques. S is the analytical hippocampal area. 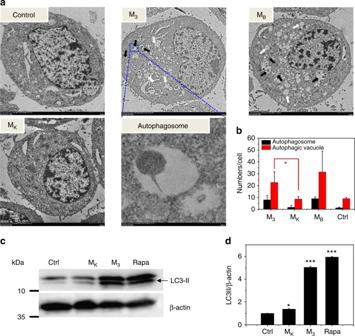Fig. 5 M3activated autophagy significantly in vitro.aTEM images of N2a cells. The N2a cells were treated with PBS (control), MK(200 μg/mL) and M3(200 μg/mL), and MB(200 μg/mL). The autophagic structures are indicated by black arrows (autophagosome), and white arrows (autophagic vacuoles).bThe static results of autophagic structures were obtained from three random TEM images. Data are presented as mean ± s.d. (n= 3).cWestern blot of LC3-II and (d) the corresponding quantified results. N2a cells were treated for 24 h with PBS (control), MK(200 μg/mL), M3(200 μg/mL), and Rapa (1 μM). Data are presented as mean ± s.d. (n= 3). Statistical significance is indicated as *p< 0.05, **p< 0.01, and ***p< 0.001, for comparison with control group (Student’st-test) For Nissl staining, half sections were stained with cresyl violet for Nissl body staining in the neurons. The sections were examined and photographed under a microscope (Nikon Eclipse E100) with DS-U3 DS Camera Control Unit. The number of staining cells was counted at 400× magnification in blinded manner, only structures of appropriate size and shape were demonstrated clearly. 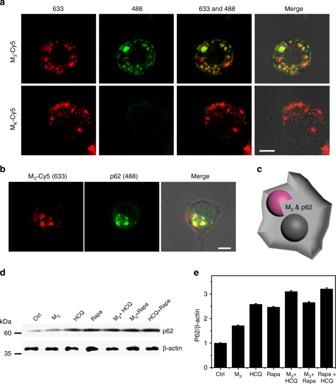Fig. 6 M3induced autophagic degradation in vitro.aCLSM images showed the co-localization of the autophagosome (GFP-LC3-positive puncta, green signals) and M3-Cy5 (red signals). N2a/GFP-LC3 cells were treated with M3-Cy5 (200 μg/mL) and MK-Cy5 as a control for 24 h.bCLSM images showed the co-localization of M3-Cy5 (red signals) and p62 (green signals from anti-p62-labeled secondary antibody).cThe schematic illustration of M3degradation by autophagy.dWestern blot of p62 and (e) the corresponding quantified results. N2a cells were cultured as follows: in regular culture medium for 24 h (lane 1); M3(200 μg/mL) for 24 h (lane 2); 5 μM HCQ for 1 h (lane 3); 1 μM Rapa for 1 h (lane 4); with M3(200 μg/mL) and HCQ (lane 5); with M3(200 μg/mL) and Rapa (lane 6); with Rapa and HCQ (lane 7). Data are presented as mean ± s.d. (n= 3). Scale bar in (a,b) is 10 µm The final results were shown as mean ± SD ( n = 6). Statistical analysis All data are reported as mean ± standard deviation (s.d.). The in vitro experiments were performed in three independent experiments with at least three technical replicates. The in vivo experiments were performed with 3–4 mice for each group. Statistical analysis of the samples was performed using Student’s t-test, and P value of <0.05 was considered significant. 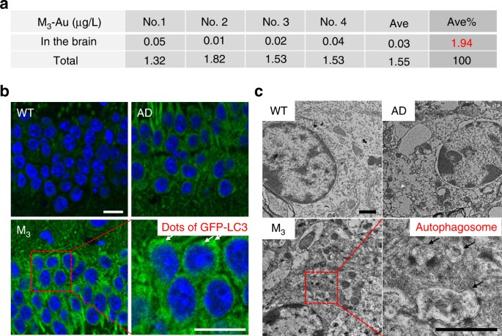Fig. 7 In vivo evaluation of M3crossing BBB and activating autophagy.aThe concentration of Au in the brain and in the total injection solution, respectively. The amount of M3actually reached to the brain was evaluated by Au amount: M3% = 0.03/1.55 × 100% = 1.94%.(n= 4).bCLSM images andcbio-TEM images of brain tissue slices of AD mice treated by PBS or M3, and WT mice treated with PBS as a control. The dots of GFP-LC3 (white arrow inb) and the strucuture of autophagsome (black arrow inc) were pointed out in M3treated AD mice, respectively. Scale bar in (b) is 20 µm. Scale bar in (c) is 1 µm 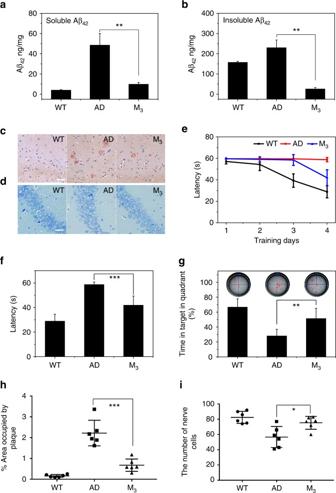Fig. 8 In vivo evaluation of M3for the clearance of Aβ and decreasing cytotoxicity.aSoluble Aβ42and (b) insoluble Aβ42in the brain measured by ELISA. (n= 4).cThe immunohistochemical analysis of Aβ42deposition in the brains of WT control mice, AD control mice, AD mice treated with M3. The Aβ42deposits appeared as brown signals as indicated by red dotted circle. Scale bar is 50 µm.dThe Nissl staining of nerve cells in the brains of WT control mice, AD control mice, AD mice treated with M3. The Nissl bodies were stained blue. Scale bar is 50 µm.eThe latencies of WT control mice, AD control mice, and AD mice treated with M3(three mice per group).fThe latency during the memory test in the MWM probe trial without a platform.gThe percent (%) of time in the targeted quadrant where the platform had been located during the memory test in the MWM probe trial.h,iwere the quantified results of (c,d), respectively. Data are presented as mean ± s.d. (n= 6). The data between AD group and M3group are analyzed by a Student’st-test. Statistical significance is indicated as *p< 0.05, **p< 0.01, and ***p< 0.001 Data availability The data that support the findings of this study are available within the article, its Supplementary Information files and from the corresponding author upon reasonable request.